A general approach to crystalline and monomodal pore size mesoporous materials Mesoporous oxides attract a great deal of interest in many fields, including energy, catalysis and separation, because of their tunable structural properties such as surface area, pore volume and size, and nanocrystalline walls. Here we report thermally stable, crystalline, thermally controlled monomodal pore size mesoporous materials. Generation of such materials involves the use of inverse micelles, elimination of solvent effects, minimizing the effect of water content and controlling the condensation of inorganic frameworks by NO x decomposition. Nanosize particles are formed in inverse micelles and are randomly packed to a mesoporous structure. The mesopores are created by interconnected intraparticle voids and can be tuned from 1.2 to 25 nm by controlling the nanoparticle size. Such phenomena allow the preparation of multiple phases of the same metal oxide and syntheses of materials having compositions throughout much of the periodic table, with different structures and thermal stabilities as high as 800 °C. The seminal introduction of MCM-41 and M-41S mesoporous materials by Mobil researchers over 20 years ago has led to tens of thousands of research projects [1] . Since this time, variations of the Mobil process have produced various new mesoporous materials, doped materials, different compositions and unique synthetic modifications such as replicas of various systems [2] , [3] , [4] . These syntheses have focused on the use of water or water plus a base, or water plus an acid or a chemical that varies the pH during the reaction with materials such as urea. Various charged ( S + or S − ) or neutral surfactants ( S 0 ), or a combination of these surfactants are used. There are either strong Coulombic interactions ( S + I − , S − I + , S + X − I + and S − X + I − ) or strong ligand–metal interactions via hydrogen bonding or coordination-type interactions, and such systems have limited thermal stabilities and mostly amorphous walls, where I is an inorganic species and X is a mediator [5] , [6] , [7] , [8] , [9] , [10] . Such syntheses are open to air with various aging times and environmental conditions that can influence the porosity of these materials. Most studies of mesoporous transition metal oxide (MTMO) materials have focused on groups I–IV, including Y, Ti, Hf, Zr, V, Nb, Ta, Cr, Mo and W [6] , [7] , [11] , [12] , [13] , [14] , [15] , [16] . Sol-gel chemistry of these transition metals (TMs) can be controlled in alcoholic solutions with proper acidity adjustments, and such metals interact strongly with polyethylene oxide (PEO) groups of non-ionic surfactants by accepting electron density to their empty d -orbitals [17] . Such control and interactions do not exist for late TMs. Mesoporous materials synthesized by the use of a soft template have low-angle X-ray diffraction peaks, indicating a meso-order and type-IV N 2 adsorption isotherms, indicating a regular mesopore structure. Water content is a critical parameter with porous TM oxide syntheses [18] , [19] . Water competes with PEO groups of non-ionic surfactants and other alkoxy groups (from solvent or precursor) for coordination to the metal centre. When excess water is used, these systems suffer from weak surfactant–TM (S–I) interactions and uncontrolled hydrolysis and condensation of inorganic sols. As most syntheses are open to the air, the water content is very difficult to control, unless a humidity chamber is employed. Therefore, when the number of water molecules per metal atom (H) is >1, phase separation and non-porous oxides are obtained [19] . On the other hand, water is essential for hydrolysis and condensation reactions, and is also important for controlling the reaction rates. When H is <1, ordered mesoporous materials are formed where the metal has empty d -orbitals to interact with solvents and surfactants [19] . These materials obtain water from the environment during synthesis or controlled amounts are intentionally added under controlled environments. When H is <<1, strong S–I interactions occur with weak surfactant–surfactant (S–S) interactions and the resulting materials are either non-porous or do not have a regular mesopore structure [19] . Thermodynamic interactions in such syntheses and factors influencing each term are given in equation 1, where Δ G m is the formation energy of the mesostructured material, Δ G org is the S–S interaction, Δ G I is the inorganic–inorganic (I–I) interaction, Δ G inter is the S–I interaction and Δ G sol is a contribution from solvent involved interactions [19] , [20] . Poor control of the last two terms, Δ G inter and Δ G sol is the main reason why conventional approaches cannot be used for later TMs. Therefore, filled or half-filled d -orbitals, such as in systems containing Mn, Fe, Co and others, are difficult to make with other methods, as charge-transfer reactions do not occur and these metals are known to not have ideal sol-gel chemistry [19] . The objective of our synthetic strategy concerns minimization of the effect of Δ G inter and Δ G sol parameters by carrying all reagents into inverse micelles to make well-ordered MTMO materials. Hydrolysis and condensation of the oxo-clusters (Δ G I ) in the inverse micelles are controlled by unique NO x chemistry formed in situ by the thermal decomposition of nitrate ions. The resulting materials are monodispersed nanoparticle aggregates and the mesopores are the connected intraparticle voids. The structural parameters (unit cell, pore size and pore volume) and crystallinity of the resulting mesoporous materials can be tuned by heat treatment cycles. The method is generic and allows one to synthesize mesoporous oxide materials from different parts of the periodic table, such as late TMs (Mn, Co, Fe and Ni), early TMs (Ti and Zr), lanthanides (Ce), metalloids (Si) and non-metals (C). Synthetic approach and characterization of reaction gel Our sol-gel-based inverse micelle method ( Fig. 1 ) uses HNO 3 at low pH to hinder condensation; metal oxo-clusters are stabilized and the clusters are confined in hydrated inverse micelles and interact with surfactant via hydrogen bonding. The surfactant species is P123; inverse micelles formed by surfactant species serve as nanoreactors and individual surfactant molecules in inverse micelles also form a physical barrier between the oxo-clusters, preventing uncontrolled aggregation. An interface modifier such as 1-butanol (for both polyethylene oxide (PEO) and polypropylene oxide (PPO)) compensates for the decrease of the aggregation number, hinders the condensation by forming a physical barrier between the oxo-clusters and limits oxidation of surfactant molecules (by TM clusters) present in the micelle. The hydrotropic nitrate ion increases solubility of P123, penetrates into the micelle and decreases the aggregation number, pulls the positively charged metal oxide clusters into the micelle and hydrates the core [21] . The existence of NO 3 − ions in the developed method is essential and such ions have multiple roles. One important role arises from the unique chemistry of nitrate ions. Thermal decomposition of nitrate ions forms a wide range of chemicals referred to as NO x [22] , [23] . Formation of NO x changes the colour of the gel to yellow (~60 min). The formed NO x species coordinate to oxo-clusters, which can be realized from the five sharp absorption bands in the region of 320–400 nm ( Fig. 2a ). The disappearance of colour in the next 30 min is followed by a quick increase in pH and formation of mesoporous oxides, as decomposition of NO x quickly consumes H + in this environment. To validate the role of NO x chemistry, a set of control experiments were conducted. For these experiments, two reaction gels were prepared by leaving out surfactant or the metal source. In the absence of metal source, NO x formation (yellow gel) indicated by five sharp absorption bands in the 320–400 nm region was not observed. Instead, only a broad absorption peak was seen ( Supplementary Fig. S1a ). On the other hand, the five absorption bands were observed for surfactant-free gel, despite the resulting final material being non-porous. Formation and disappearance of the yellow colour and also formation of the mesoporous oxides on decolourization of the gel are observed in other studied systems. Supplementary Fig. S1b,c show the ultraviolet–visible spectra of the reaction gels of mesoporous cobalt and nickel, respectively. The reaction gels show the characteristic sharp absorption bands originating from NO x adsorption on metal oxo-clusters. The formation of coordinated nitrate species on coordination of NO x on oxo-clusters is also confirmed by attenuated total reflectance Fourier transform infrared (ATR–FTIR) spectroscopy ( Supplementary Fig. S1d ) [22] , [24] . 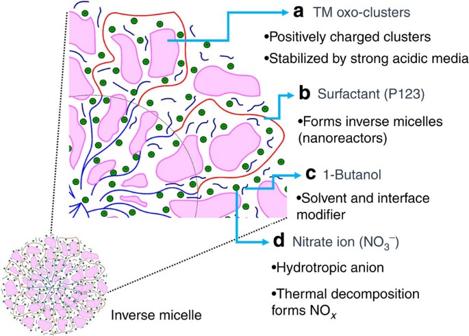Figure 1: Inverse micelle sol-gel method and roles of components. (a) TM oxo-clusters: positively charged oxo-clusters interact with surfactant via hydrogen bonding and the charge is balanced by negatively charged nitrate ions (NO3−). (b) Surfactant (P123): inverse micelles are formed by P123 (EO20–PPO70–PEO20) surfactant. Later, the inverse micelles are packed to form the material. (c) 1-Butanol: solubilizes the surfactant (solvent) and stabilizes inverse micelles (modifier). (d) Nitrate ion (NO3−): hydrotropic nitrate anion penetrates into the core of inverse micelles to hydrate it and pulls positively charged oxo-clusters into the micelles. Thermal decomposition of nitrate ions form nitric oxides (NOx) to control the sol-gel chemistry. Formed NOxis adsorbed on oxo-clusters to hinder uncontrolled condensation. Figure 1: Inverse micelle sol-gel method and roles of components. ( a ) TM oxo-clusters: positively charged oxo-clusters interact with surfactant via hydrogen bonding and the charge is balanced by negatively charged nitrate ions (NO 3 − ). ( b ) Surfactant (P123): inverse micelles are formed by P123 (EO 20 –PPO 70 –PEO 20 ) surfactant. Later, the inverse micelles are packed to form the material. ( c ) 1-Butanol: solubilizes the surfactant (solvent) and stabilizes inverse micelles (modifier). ( d ) Nitrate ion (NO 3 − ): hydrotropic nitrate anion penetrates into the core of inverse micelles to hydrate it and pulls positively charged oxo-clusters into the micelles. Thermal decomposition of nitrate ions form nitric oxides (NO x ) to control the sol-gel chemistry. Formed NO x is adsorbed on oxo-clusters to hinder uncontrolled condensation. 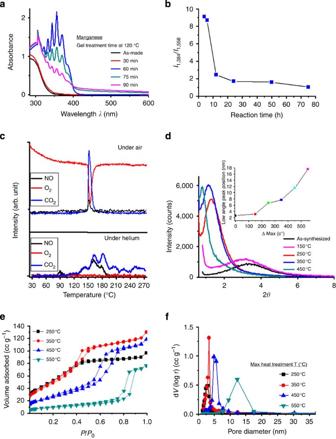Figure 2: Characterization of the reaction gel and materials. (a) Ultraviolet–visible spectra of mesoporous manganese oxide reaction gel heated at 120 °C for 0–90 min. (b) Normalized FTIR intensity ratio ofIν1of NO3−(at 1,384 cm−1) andIνasof R-COO−(at 1,558 cm−1) of solvent-extracted samples synthesized at different reaction times. (c) TPD of as-synthesized mesoporous manganese oxide sample under air and helium flow (50 cc min−1) in 30–275 °C region. (d) Low-angle PXRD and low-angle peak positions (nm), (e) N2sorption isotherms and (f) BJH desorption pore-size distributions of mesoporous manganese oxide (Meso-Mn-X) samples heat treated at different final temperatures. Full size image Figure 2: Characterization of the reaction gel and materials. ( a ) Ultraviolet–visible spectra of mesoporous manganese oxide reaction gel heated at 120 °C for 0–90 min. ( b ) Normalized FTIR intensity ratio of I ν1 of NO 3 − (at 1,384 cm −1 ) and I νas of R-COO − (at 1,558 cm −1 ) of solvent-extracted samples synthesized at different reaction times. ( c ) TPD of as-synthesized mesoporous manganese oxide sample under air and helium flow (50 cc min −1 ) in 30–275 °C region. ( d ) Low-angle PXRD and low-angle peak positions (nm), ( e ) N 2 sorption isotherms and ( f ) BJH desorption pore-size distributions of mesoporous manganese oxide (Meso-Mn- X ) samples heat treated at different final temperatures. Full size image During this process, surfactant species are oxidized at long reaction times and form carboxyl groups coordinated to metal oxygen clusters and compete with nitrate to exist in the micelles. Therefore, during the synthesis, carboxylate bands increase whereas nitrate-related bands decrease. The relative ratio of spectra (normalized with respect to the Mn–O stretching band (584 cm −1 )) confirms that reaction times longer than 6 h ( t >6 h) result in oxidation of surfactant to form carboxyl groups ( Fig. 2b and Supplementary Fig. S2a ) here for manganese-based systems. These samples ( t >6 h) show thermal stabilities up to 250 °C, whereas samples at t < 6 h have a thermal stability up to 550 °C (based on the disappearance of the low-angle diffraction line). The carboxyl groups and nitrates formed on as-synthesized manganese oxide samples are oxidized and removed at 150 °C ( Supplementary Fig. S2b ). Nitrate ions do not fully disappear until 250 °C. The carboxyl and nitrate removal was also monitored by temperature-programmed desorption (TPD) studies under air and He flows ( Fig. 2c ). The carboxyl groups leave the surface as CO 2 and nitrate groups leave the surface as NO in the temperature range of 150–170 °C under air flow. However, under helium flow, desorption of CO 2 and NO are slower and occur at higher temperatures. Moreover, the powder X-ray diffraction (PXRD) pattern of used material (under He flow) shows the Mn 3 O 4 phase, suggesting reduction of manganese species by carboxyl and nitrate removal ( Supplementary Fig. S2c ). The mesostructured manganese materials with Mn 3 O 4 phase are not thermally stable and the low-angle diffraction line disappears at temperatures above 250 °C. Therefore, the carboxyl and nitrate removal is complete under heat treatment in air. The process of carboxyl and nitrate removal was also monitored for other metal systems mentioned in the manuscript (Fe, Co and Ni) ( Supplementary Fig. S3 ). TPD and FTIR data show very similar desorption profiles, and for all metal systems carboxyl and nitrate species are removed in the 150–190 °C temperature range. The carboxyl groups are mostly removed by heating the as-synthesized materials at 150 °C for 12 h and followed by heating at 250 °C for 1–4 h. The removal process was also followed by recording FTIR spectra of the powders at different time intervals during the heating process ( Supplementary Fig. S3b–d ). The carboxyl groups and nitrate ions need to be mostly removed before proceeding with further heat treatment to preserve the mesoporous structure. Failure to remove the carboxylate groups and nitrate ions leads to thermally unstable mesoporous materials. Supplementary Fig. S4 shows the (a) low-angle PXRD, (b) wide-angle PXRD and (c) N 2 sorption isotherms of as-synthesized mesoporous samples directly heated to 250 °C for 4 h without 150 °C heat treatment. All samples show no or very weak low-angle diffraction lines, and all show non-porous features in N 2 analyses along with very low Brunauer-Emmett-Teller (BET) surface areas. Physicochemical properties of mesoporous TM oxides A typical ordered mesoporous material is characterized by a low-angle diffraction line(s), indicating the existence of a mesostructure and a type-IV adsorption isotherm, indicating a regular nanosized pore structure. In addition, trends of both mesopore sizes and unit cell parameters on template removal (by calcination) or heat treatment owing to further condensation of the inorganic walls contradict literature reports. A remarkable observation is that during thermal treatment both the d -spacings and the pore sizes increase for inverse micelle-templated mesoporous materials. Figure 2d shows the low-angle diffraction lines for mesoporous manganese oxide (Meso-Mn- X , where X =150–550 °C) samples heated to different final temperatures. The low-angle diffraction line position gradually shifts from 3.1 to 17.5 nm (unit cell expansion) by increasing the final heat treatment temperature from 150 to 450 °C ( Table 1 ). Similarly, Barrett-Joyner-Halenda (BJH) desorption pore diameters increase (from 2.0 to 12.5 nm) with the heat treatment, and regardless of the heat-treatment temperature the materials show characteristic type-IV adsorption isotherms, suggesting the materials preserve the mesoporous structure ( Fig. 2e ). Corresponding BET surface areas (100–260 m 2 g −1 ), pore-size distributions and pore volumes (up to 0.22 cc g −1 ; Fig. 2c–e and Table 1 ) show that these mesporous materials are produced with excellent control of pore-size distributions. Such control of pore-size distribution, enhanced pore volumes and thermal stabilities are unprecedented with TM oxide mesoporous materials [25] . Wide-angle PXRD patterns of the mesoporous manganese oxide (Meso-Mn- X , X =150–550 °C) samples heated to different final temperatures are given in Supplementary Fig. 5Sa and Table 1 . The materials are amorphous at low temperatures (150–350 °C) and become crystalline with the bixbyite (Mn 2 O 3 ) phase at high temperatures (450 and 550 °C). Two other phases obtained with mesostructures (based on the existence of low-angle diffraction lines) are Hausmannite (Mn 3 O 4 ) and Manganite (MnOOH) phases, which were obtained at long reaction times ( Supplementary Fig. 5Sb–e ). 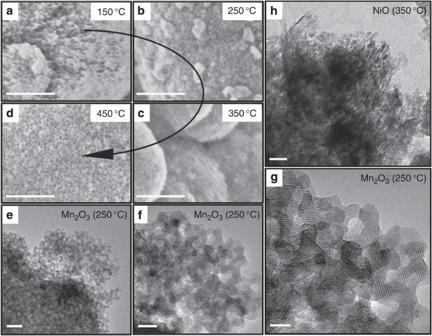Figure 3: Electron microscopy images. FESEM images of mesoporous Mn2O3after heat treatments at different temperatures: (a) 150, (b) 250, (c) 350 and (d) 450 °C, (scale bars, 200 nm). HR-TEM images of (e) Meso-Mn-250 (scale bar, 20 nm), (f) Meso-Mn-250 (scale bar, 10 nm), (g) Meso-Mn-250 (scale bar, 5 nm) and (h) Meso-Ni-350 (scale bar, 20 nm). Figure 3a–d shows field-emission scanning electron microscopy (FESEM) images for mesoporous manganese oxides at various stages of thermal treatment in the syntheses, showing development of pores. At 450 °C, uniform pores are observed in these FESEM images all over the material. The transmission electron microscopy (TEM) data of mesoporous manganese oxide and nickel oxide ( Fig. 3e–h , respectively) are also typical of all these materials and show that these systems are made of small crystalline nanosize particles that are organized and that remain stable even with thermal treatments at elevated temperature (550 °C for manganese). The nanoparticle sizes and enhancements in pore size were also monitored for mesoporous manganese systems heated to different final temperatures with TEM. 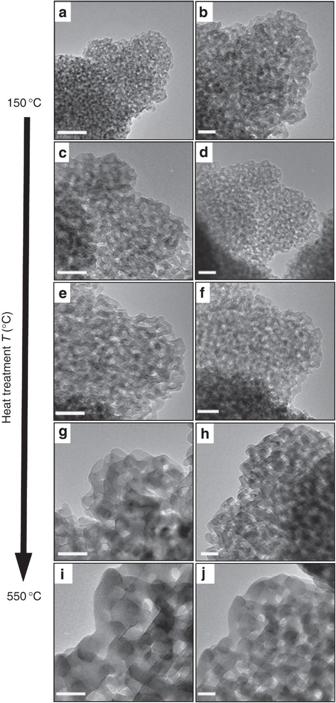Figure 4: HR-TEM images showing pore expansion and particle growth. HR-TEM images of mesoporous manganese oxide at different final heat treatment temperatures: (a) 150, (b) 150, (c) 250, (d) 250, (e) 350, (f) 350, (g) 450, (h) 450, (i) 550 and (j) 550 °C (scale bars, 20 nm). Figure 4 shows the TEM images of mesoporous manganese oxide from the same experimental batch and heated to different final temperatures. All TEM images are collected with the same magnifications; hence, the progressive growth of both the pore size and nanoparticles with temperature increase can be readily observed. Table 1 Structural parameters of mesoporous materials discussed in the manuscript. Full size table Figure 3: Electron microscopy images. FESEM images of mesoporous Mn 2 O 3 after heat treatments at different temperatures: ( a ) 150, ( b ) 250, ( c ) 350 and ( d ) 450 °C, (scale bars, 200 nm). HR-TEM images of ( e ) Meso-Mn-250 (scale bar, 20 nm), ( f ) Meso-Mn-250 (scale bar, 10 nm), ( g ) Meso-Mn-250 (scale bar, 5 nm) and ( h ) Meso-Ni-350 (scale bar, 20 nm). Full size image Figure 4: HR-TEM images showing pore expansion and particle growth. HR-TEM images of mesoporous manganese oxide at different final heat treatment temperatures: ( a ) 150, ( b ) 150, ( c ) 250, ( d ) 250, ( e ) 350, ( f ) 350, ( g ) 450, ( h ) 450, ( i ) 550 and ( j ) 550 °C (scale bars, 20 nm). Full size image Pore expansion and increase in d -spacing with thermal treatments were also observed in other TM systems (iron (Meso-Fe- X ), cobalt (Meso-Co- X ) and nickel (Meso-Ni- X ). Low- and wide-angle PXRD patterns, N 2 sorption isotherms, BJH desorption pore-size distributions, FESEM and TEM images of mesoporous iron (meso-Fe- X ), cobalt (meso-Co- X ) and nickel (meso-Ni- X ) are demonstrated in Supplementary Figs S6–S8 , respectively. The temperature (heat treatment)-dependent unit cell increase (a decrease in the low-angle diffraction line position) and pore expansion were also observed for these materials. As in the manganese system (meso-Mn), High-resolution transmission electron microscopy (HR-TEM) images for other mesoporous materials also demonstrate the nanoparticle aggregate nature of these mesoporous materials. The thermal stabilities of these materials are similar to the manganese system, and the mesostructure (low-angle diffraction line) disappears at 500, 400 and 500 °C for iron, cobalt and nickel systems, respectively. The heat-treatment temperatures reported in Table 1 are the final temperatures for each material and any further temperature increase results in disappearance of the mesostructure. There are several advantages of this method, including control of the crystal structure of the wall during heating, precise control of pore size and, most importantly, the method has been demonstrated to work for synthesizing numerous mesoporous oxides. The generality of the approach is illustrated for various oxide materials from different parts of the periodic table, which are shown in Supplementary Figs S9 to S14 and Supplementary Table S2 . One TM from group IV (Zr), one TM from group V (Nb), one post-TM (Sn), one lanthanide (Ce), one mixed metal (yttria stabilized zirconia (YSZ)) and one TM chalogenide (CdS) are used to demonstrate the generality of the approach. For the syntheses of mesoporous Si and Zr alkoxide sources were used, and chloride sources were used in the Nb system. Such data show that the method is not limited only to nitrate sources. However, using sulphate sources results in cloudy gels or surfactant precipitation out of the gel. As the main nitrate source is nitric acid, enough nitrate ions are still present in the reaction gel when non-nitrate sources are used. Different from the late TMs (Mn, Fe and Co), the adsorbed NO x and carboxyl species on the surface of as-synthesized materials are not a concern for these systems, as they do not have the possibility of forming multiple oxidation states. Therefore, these materials were directly calcined at a target temperature for a certain time (see Methods section). All materials show one characteristic low-angle diffraction line and the position of the line shifts to lower angles with increased heat treatment ( Supplementary Figs S9–S14a and Supplementary Table S2 ). Most samples show characteristic type-IV adsorption isotherms, indicating the existence of a mesoporous structure ( Supplementary Figs S9–S14c ). The obtained pore-size distributions for these materials are given in Supplementary Table S2 . Electron microscopy images suggest that the materials are in the form of crystalline nanoparticle aggregates, see Supplementary Fig. S9f (Meso-Zr), Supplementary Fig. S11e (Meso-Sn) and Supplementary Fig. S12e (Meso-Ce). Nanocasting and bifunctional catalysis One of the important applications of mesoporous materials with different mesostructures and mesoporosities is their use as a hard template (nanocasting) for the synthesis of mesoporous carbon materials [26] , [27] , [28] . Porous carbon materials have been used in a variety of fields such as electrode materials, fuel cell electrodes, capacitors, separations and catalysis [27] , [28] . In addition, the entire process also gives vital information about the nature of the mesoporous template [27] . For example, preserving the mesoporosity of the synthesized carbon materials by nanocasting depends on the existence of interconnecting channels in the templated porous material [27] . 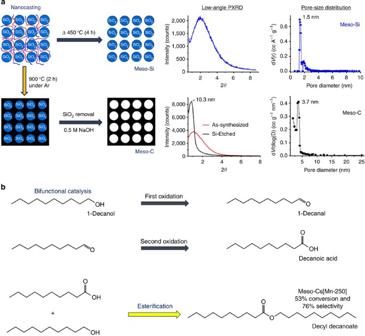Figure 5: Some unique properties of inverse micelle template mesoporous materials. (a) Illustration of the formation mechanism of mesoporous carbon (Meso-C) by nanocasting microporous silica (Meso-Si) along with low-angle PXRD and pore-size distribution graphs. (b) Reaction pathway of double oxidation of 1-decanol to decanoic acid, and then followed by an esterification reaction between 1-decanol andin-situ-formed decanoic acid to form decyl decanoate with mesoporous manganese oxide samples (Meso-Mn-250 and Meso-Cs[Mn-250]), OMS-2, amorphous manganese oxide and commercial Mn2O3. Figure 5a shows the schematic description of the nanocasting approach along with the low-angle PXRD diffractions and pore-size distributions of the mesoporous silica template (Meso-Si) and carbon material (Meso-C). The formed carbon materials preserve the mesoporosity and mesostructure, indicating the existence of interconnecting channels in synthesized Meso-Si materials. Figure 5: Some unique properties of inverse micelle template mesoporous materials. ( a ) Illustration of the formation mechanism of mesoporous carbon (Meso-C) by nanocasting microporous silica (Meso-Si) along with low-angle PXRD and pore-size distribution graphs. ( b ) Reaction pathway of double oxidation of 1-decanol to decanoic acid, and then followed by an esterification reaction between 1-decanol and in-situ -formed decanoic acid to form decyl decanoate with mesoporous manganese oxide samples (Meso-Mn-250 and Meso-Cs[Mn-250]), OMS-2, amorphous manganese oxide and commercial Mn 2 O 3 . Full size image These mesoporous materials also show excellent catalytic activities and stabilities in various reactions and Fig. 5b illustrates one of these. Meso-Mn-250- and Cs-promoted mesoporous manganese oxide (Meso-Cs[Mn-250]) were used to oxidize an aliphatic alcohol (1-decanol) twice (first to 1-decanal and then to decanoic acid) and then to decanoic acid ester (decyl decanoate) by esterification reactions under mild reaction conditions (under air reflux). The first two reactions show the oxidation power of the catalyst. Oxidation of aliphatic alcohols to carboxylic acids can only be done in the presence of strong oxidants (peroxide or molecular O 2 under high pressure) and mostly with noble metal catalysts [29] , [30] . The second reaction shows the basic nature of the catalyst [29] , [31] . To date, such a set of reactions has not been observed with TM oxide catalysts and with such mild conditions (air as oxidant and under ambient pressure). Supplementary Table S3 shows the conversions and selectivities to three products. The meso-Mn-250 sample shows a relatively high conversion (as high as 22%) and selectivity towards 1-decanal (100%); however, its non-porous counterpart (commercial Mn 2 O 3 ) shows no activity for 1-decanol oxidation. When compared with ion-promoted state-of-the-art manganese oxide catalysts (OMS-2 and amorphous manganese oxide), meso-Mn-250 is still more active for 1-decanol oxidation ( Fig. 5b ). Ion (Cs)-promoted mesoporous manganese oxide (Meso-Cs[Mn-250]) showed the best activity among the catalysts tested and conversion reached 53% with a decyl decanoate selectivity of 23% (and 76% decanoic acid). The other ion-promoted manganese oxide catalysts (OMS-2 and amorphous manganese oxide) can only do one-step oxidations to aldehyde. However, Meso-Cs[Mn-250] can oxidize 1-decanol first to 1-decanal and then to decanoic acid. Next, this catalyst further converts decanoic acid to decyl decanoate by esterification reactions between decanoic acid and 1-decanol. Our hypothesis is that careful control of the reaction medium and reagents allows preparation of well-ordered crystalline TM oxide materials that are markedly different from the traditional silica-based synthetic routes and original mechanisms (( S + I − , S − I + , S + X − I + and S − X + I − ) proposed in the literature [6] , [7] , [8] , [9] . Silica has limited structures under normal mesoporous synthetic conditions, whereas TM oxides are well known to have multiple structures in the temperature range of 25 to 800 °C [10] . There should be other general synthetic mechanisms to prepare MTMO materials than traditional routes. In these syntheses, the effect of key thermodynamic parameters Δ G inter (everything is in the micelle) and Δ G sol (no solvent effects in the inverse micelle) are minimized. In addition, Δ G I is controlled by making the entire reaction occur in inverse micelles, and unique NO x chemistry and Δ G org are adjusted with NO 3 − and 1-butanol. The materials synthesized with this approach result in mesoporous materials that have markedly different structural properties than materials prepared by traditional approaches. According to our model, the low-angle peak position corresponds to the average sizes of the building blocks (nanoparticles) and the mesopores are formed by connected intraparticle voids. Therefore, unit cell expansion during heat treatment signifies an increase in nanoparticle size (nanoparticles sinter to form bigger ones) with a concomitant increase in size of intraparticle voids (mesopores). We are not aware of this phenomenon previously being observed for reported mesoporous materials. Unlike mesoporous materials by inverse micelle packing method, conventional mesoporous materials reported in the literature on heat treatment (calcination) show a decrease in pore size owing to further condensation of mesopore walls. The exact position of the low-angle peak in these mesoporous materials depends on the heating temperature and time, and the material being studied. A proposed formation mechanism of the ordered mesopores is shown in Fig. 6 . First, metal precursor-loaded inverse micelles are packed on solvent removal; packing is followed by oxidation and condensation of the metal precursors in the micelles. Finally, the surfactants are washed off, and surface NO x and carboxyl species are removed at 150 °C for 12 h followed by a second heating step at 250 °C for 1–4 h. Mesopores merge to form larger-ordered mesoporous materials during the heating cycles. The crystalline walls are made up of nanoparticles of metal oxides that order as observed by PXRD, HR-TEM and electron diffraction methods. Meso-order (low-angle PXRD) and mesoporosity (type-IV adsorption isotherms) are both formed by packing of nano oxide particles. The mesopores are the intraconnecting voids formed in between randomly packed nanocrystals. Formation of microporosity and mesoporosity by aggregation of colloidal nanoparticles or using these materials for nanocasting has previously been observed [32] . 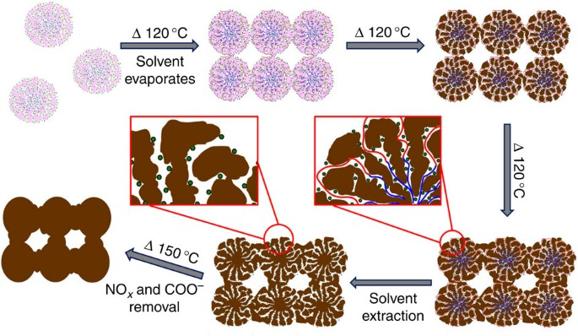Figure 6: Proposed formation mechanism of inverse micelle-templated mesoporous materials. Formed inverse micelles are packed and then inorganic component is condensed and oxidized. Surfactants are removed by ethanol washing (solvent extraction) and adsorbed species (NOxand COO−) are removed by a heat treatment at 150 °C (12 h). Figure 6: Proposed formation mechanism of inverse micelle-templated mesoporous materials. Formed inverse micelles are packed and then inorganic component is condensed and oxidized. Surfactants are removed by ethanol washing (solvent extraction) and adsorbed species (NO x and COO − ) are removed by a heat treatment at 150 °C (12 h). Full size image In summary, a general approach for the synthesis of mesoporous metal oxides is introduced. This approach allows synthesis of mesoporous materials from different parts of the periodic table. There are several advantages of the approach over traditional methods such as the following: H is not a concern; in principle, the method is applicable to all TMs; gel aging is not required; various crystal structures can be formed; thickness of walls can be controlled (by controlling the size of nanoparticles); and this is the first time pore expansion on heat treatment of MTMO materials has been observed. Over 60 new mesoporous materials with tunable porosity and crystallinity have been synthesized with the current approach. These mesoporous materials have unique stability, structural and porous properties that can be readily tailored for different applications. Extensions of this study to other mesoporous materials and their applications in various fields are underway. Chemicals Manganese (II) nitrate tetrahydrate (Mn(NO 3 ) 2 .4H 2 O, ≥97.0), iron (III) nitrate nonahydrate (Fe(NO 3 ) 3 .9H 2 O, ≥98.0), cobalt (II) nitrate hexahydrate (Co(NO 3 ) 2 .6H 2 O, ≥98.0), nickel (II) nitrate hexahydrate (Ni(NO 3 ) 2 .6H 2 O, ≥98.5), tetraethylorthosilicate (≥99.0), zirconium (IV) butoxide solution (80wt% in 1-butanol), cerium (III) nitrate hexahydrate (Ce(NO 3 ) 3 .6H 2 O, 99%), tin (IV) tert-butoxide (Sn(OC(CH 3 ) 3 ) 4 , ≥99.99), niobium (V) chloride (NbCl 5 , 99%), thiourea (≥99%), cadmium nitrate tetrahydrate (Cd(NO 3 ) 2 .4H 2 O, 98%), yttrium (III) nitrate hexahydrate (Y(NO 3 ) 3 .6H 2 O, 99.8%), 1-butanol (anhydrous, 99.8%) and Poly (ethylene glycol)-block-Poly(propylene glycol)-block-Poly(ethylene glycol) PEO 20 –PPO 70 –PEO 20 (Pluronic P123) were all purchased from Sigma-Aldrich. Concentrated nitric acid (HNO 3 , 68–70%) was purchased from J.T. Baker. All chemicals were used as received and used without further purification. Manganese oxides OMS-2 and amorphous manganese oxides were synthesized by methods reported in the literature [33] , [34] . Synthesis of mesoporous first-row TM oxides The inorganic source (0.01–0.02 mol) was dissolved in a solution containing 0.188–0.27 mol of 1-butanol, 0.032–0.038 mol of HNO 3 and 2.04–4.08 × 10 −4 mol of P123 surfactant in a 150-ml beaker at room temperature (RT) and under magnetic stirring. The obtained clear gel is placed in an oven at 95–120 °C for 2–6 h. The obtained powder is washed several times with ethanol and then the powder is centrifuged. Finally, the powder is dried in a vacuum oven overnight. The dried powders are subjected to heating cycles to achieve desired crystal structure and mesopore size. Supplementary Table S1 shows the concentrations and reaction conditions used for each different metal system studied, as well as the heating cycles applied. Heating cycles are needed to apply starting from the lowest temperature. For example, to heat a sample to 550 °C, first the material is heated to 150 °C for 12 h+250 °C for 3–4 h+350 °C for 2–3 h+450 °C for 1–2 h. The powder is naturally cooled down to RT after each heating step. All heat treatments were done under air. The samples are labelled as Meso-M- X , where M is the TM (such as Mn and Fe) and X is the final heating temperature. Synthesis of mesoporous silica Tetraethylorthosilicate (0.02 mol) was diluted in a solution containing 0.188 mol (14 g) of 1-butanol, 0.032 mol (2 g) of HNO 3 and 3.4 × 10 −4 mol (2 g) of P123 surfactant in a 150-ml beaker at RT and under magnetic stirring. The obtained clear gel was placed in an oven at 120 °C for 4–6 h. The obtained transparent yellow film was placed in a calcination cuvette and calcined directly under air at 450 °C for 4 h (1 °C min −1 heating rate). Synthesis of mesoporous carbon As-synthesized mesoporous silica sample (Meso-Si) was placed in a tubular furnace and heated to 900 °C for 2 h under an Ar atmosphere. Resulting black material was put and stirred in a 0.5 M warm NaOH solution for etching out the silica to form mesoporous carbon. The formed black powder was washed several times with water and ethanol, and dried in a vacuum oven overnight. Synthesis of mesoporous zirconium oxide Zirconium (IV) butoxide (0.02 mol) was diluted in a solution containing 0.188 mol (14 g) of 1-butanol, 0.032 mol (2 g) of HNO 3 and 3.4 × 10 −4 mol (2 g) of P123 surfactant in a 150-ml beaker at RT and under magnetic stirring. The obtained clear gel was placed in an oven at 120 °C for 4–6 h. The obtained transparent greenish film was placed in a calcination cuvette and calcined directly under air at 450 °C for 4 h or 500 °C for 3 h, or 600 °C for 1 h (2 °C min −1 heating rate). Synthesis of mesoporous cerium oxide Cerium (III) nitrate hexahydrate (0.02 mol) was dissolved in a solution containing 0.188 mol (14 g) of 1-butanol, 0.032 mol (2 g) of HNO 3 and 5.1 × 10 −4 mol (3 g) of P123 surfactant in a 150-ml beaker at RT and under magnetic stirring. The obtained clear gel was placed in an oven at 120 °C for 5 h. The obtained powder was washed several times with ethanol and then the powder was centrifuged. Finally, the powder was dried in a vacuum oven overnight. The dried powders were subjected to heating cycles to achieve desired crystal structure and mesopore size. Heating cycles are needed to apply starting from the lowest temperature. For example, to heat a sample to 550 °C, first the material is heated to 150 °C for 12 h+250 °C for 4 h+350 °C for 3 h+450 °C for 1 h+550 °C for 1 h+600 °C for 1–2 h. The powder is naturally cooled down to RT after each heating step. All heat treatments were done under air. Synthesis of mesoporous tin oxide Tin (IV) tert-butoxide (0.012 mol) was diluted in a solution containing 0.134 mol (10 g) of 1-butanol and 2.6 × 10 −4 mol (1.5 g) of P123 surfactant in a 150-ml beaker at RT and under magnetic stirring. To the above gel, diluted nitric acid solution (1 g of (0.016 mol) HNO 3 +5 g of 1-butanol) was added. The formed opaque white gel was stirred at RT for 1 h and then placed in an oven at 120 °C for 4 h. The obtained white material was placed in a calcination cuvette and calcined directly under air at 450 °C for 3 h (1 °C min −1 heating rate). Synthesis of mesoporous niobium oxide Niobium (V) chloride (0.01 mol) was dissolved in a solution containing 0.201 mol (15 g) of 1-butanol, 0.032 mol (2 g) of HNO 3 and 3.4 × 10 −4 mol (2 g) of P123 surfactant in a 150-ml beaker at RT and under magnetic stirring. The obtained clear gel was placed in an oven at 120 °C for 4–5 h. The obtained thick gel was placed in a calcination cuvette and calcined directly under air at 500 °C for 1 h (2 °C min −1 heating rate). Synthesis of meszoporous yttria stabilized zirconia Zirconium (IV) butoxide (0.02 mol) was diluted in a solution containing 0.188 mol (14 g) of 1-butanol, 0.032 mol (2 g) of HNO 3 and 3.4 × 10 −4 mol (2 g) of P123 surfactant in a 150-ml beaker at RT and under magnetic stirring. To the above clear gel, 0.001 mol yttrium (III) nitrate hexahydrate was added and dissolved under magnetic stirring. The obtained clear gel was placed in an oven at 120 °C for 4–6 h. The white material was placed in a calcination cuvette and calcined directly under air at 700 °C for 1 h (2 °C min −1 heating rate). Synthesis of mesoporous Cs promoted mesoporous manganese oxide Manganese (II) nitrate tetrahydrate (0.02 mol) was dissolved in a 1-butanol solution containing 0.188 mol (14 g) 1-butanol, 0.032 mol (2 g) of HNO 3 and 3.4 × 10 −4 mol (2 g) of P123 surfactant in a 150-ml beaker at RT and under magnetic stirring. To this clear aqueous solution, 100 μl of 2.0 M CsNO 3 was added maintaining the Mn:X ratio as 100:1. The resulting clear solution was then kept in an oven at 120 °C for 3 h under air. The resulting black powder was washed with excess ethanol, centrifuged and dried in vacuum oven overnight. The dried black powder was then heated to 150 °C for 12 h and 250 °C for 3 h under air. Synthesis of mesoporous cadmium sulphide Cadmium nitrate tetrahydrate (0.02 mol) was dissolved in a solution containing 0.201 mol (15 g) of 1-butanol, 0.032 mol (2 g) of HNO 3 and 3.4 × 10 −4 mol (2 g) of P123 surfactant in a 150-ml beaker at RT and under magnetic stirring. The obtained clear gel was placed in an oven at 120 °C for 1–2 h and obtained gel was added on urea (urea:metal is 1:1), which was in a glass autoclave. The glass autoclave was sealed and placed in oven at 75 °C for 6 h. The obtained powders were washed with water and then with ethanol, and dried in a vacuum oven overnight. Characterization PXRD analyses were performed on a Rigaku Ultima IV diffractometer (Cu Kα radiation, λ =1.5406 A) with an operating voltage of 40 kV and a current of 44 mA. FTIR spectra of powder samples were collected using a Thermoscientific Nicolet 8700 spectrometer. Sixty-four scans were collected with a 4-cm −1 spectral resolution in the absorbance mode. Powder samples were diluted with KBr and pellets were pressed from the powder mixture. Ultraviolet–visible spectra of reaction gels at different time intervals were recorded by Shimadzu UV-2450 ultraviolet–visible spectrophotometer. Diffuse reflectance ultraviolet–visible spectra of the powder samples were collected with a diffuse reflectance (DR) apparatus attached on Shimadzu UV-2450 ultraviolet–visible spectrophotometer. The powder samples were diluted in barium sulphate and pressed into sample holder. ATR–FTIR spectra of reaction gels were collected by Thermoscientific Nicolet iS5 FT-IR spectrometer equipped with iD3 ATR accessory (ZnSe). For time-dependent COO- and NO x desorption studies, the samples are diluted with KBr and pelletized (133 mm diameter). FTIR spectra of the pellets were collected using a Thermoscientific Nicolet 8700 spectrometer equipped with MCT/A detector. Sixty-four scans were collected with a 4-cm −1 spectral resolution in the absorbance mode. TPD-mass spectrometry analyses were performed with a home-made setup and an MKS-UT1 PPT quadrupole mass spectrometer. One hundred milligrams of as-synthesized mesoporous material was packed in a quartz tube and the tube was placed into a horizontal tubular furnace. The loaded sample was heated from RT to 300 °C with a 5 °C min −1 heating rate under 50 s.c.c.m. air flow (or He). The tracked masses ( m/z ) are 28 (CO), 30 (NO), 32 (O 2 ), 44 (CO 2 ) and 46 (NO 2 ). Morphological characterization was done using a Zeiss DSM 982 Gemini FESEM with a Schottky emitter at an accelerating voltage of 2.0 kV and a beam current of 1.0 mA. Nitrogen sorption experiments were conducted on a Quantachrome Autosorb-1-1C automated adsorption system. The powders were degassed for 6 h before measurement. The surface area is calculated by BET method and pore size distributions are calculated by BJH method from desorption isotherm. HR-TEM images of synthesized mesoporous materials were recorded on a JEOL 2010 FasTEM microscope operating at 200 kV. Double oxidation and in-situ esterification catalytic studies 1-Decanol (1 mmol), catalyst (100 mg) and toluene (15 ml) were taken in a 50-ml two-necked round-bottom flask equipped with a condenser. The flask was immersed in a silicon oil bath preheated to 110 °C. The reaction mixture were refluxed and stirred for 15 h under air flow. The mixture was cooled after the reaction, the catalyst was removed by filtration and gas chromatography/mass spectrometry was used to analyse the filtrate. The conversion was measured by comparing the peak areas of reactant and products. The selectivity was measured as follows: (peak area of particular product/peak area of all products) × 100. How to cite this article: Poyraz, A. S. et al. A general approach to crystalline and monomodal pore size mesoporous materials. Nat. Commun. 4:2952 doi: 10.1038/ncomms3952 (2013).